Highly confined ions store charge more efficiently in supercapacitors Liquids exhibit specific properties when they are adsorbed in nanoporous structures. This is particularly true in the context of supercapacitors, for which an anomalous increase in performance has been observed for nanoporous electrodes. This enhancement has been traditionally attributed in experimental studies to the effect of confinement of the ions from the electrolyte inside sub-nanometre pores, which is accompanied by their partial desolvation. Here we perform molecular dynamics simulations of realistic supercapacitors and show that this picture is correct at the microscopic scale. We provide a detailed analysis of the various environments experienced by the ions. We pick out four different adsorption types, and we, respectively, label them as edge, planar, hollow and pocket sites upon increase of the coordination of the molecular species by carbon atoms from the electrode. We show that both the desolvation and the local charge stored on the electrode increase with the degree of confinement. Supercapacitors are electrochemical devices which store energy through reversible adsorption of ionic species on electrode surfaces [1] . The amount of electricity which can be accumulated upon charging depends mostly on the number of ionic charges that can be accommodated per unit surface area, but it is not the sole factor. In concentrated electrolytes, and even more in ionic liquids, ions interact strongly with their counterions, leading to non-trivial structural patterns for the adsorbed ionic layers [2] , [3] , thus impacting the supercapacitor performance. In particular, the overscreening effect [4] was shown to be the origin of the low capacitance of planar electrodes. Nanoporous carbons are excellent materials for supercapacitor electrodes [5] , [6] , [7] , [8] , with enhanced capacitances: owing to confinement effects, the overscreening is quenched, leading to a more efficient charge storage characterized by much higher capacitances [9] and a large electronic screening by the pore walls of like–like ions repulsive Coulombic interactions occurs, allowing for a denser packing of the ions inside the pores [10] , [11] . In fact, the generic name of ‘nanoporous carbons’ identifies a large number of families of compounds, which are synthesized by different pathways. Their structure can be regular (carbon nanotubes, nanospheres [12] ) or disordered, non-functionalized or activated, leading to a huge variety of atomic-scale environments (curvature, porosity) experienced by the ions from the electrolyte. This local structure has barely been investigated by simulation and experimental techniques, and its consequence on the supercapacitor performance remains unknown. Here we characterize via molecular dynamics simulations the various adsorption modes for ions in a disordered nanoporous carbon electrode model and we show that the local charge storage efficiency on the electrode surface is strongly correlated with the degree of confinement (DoC) of the nearby adsorbed ions. Supercapacitors simulations We have used similar supercapacitor cells to the ones described in reference [9] . They consist of an electrolyte surrounded by two porous electrodes held at constant electrical potential, the latter aspect being important for having a realistic model [13] . In this model, the local charges on the atoms of the electrode vary dynamically in response to the electrical potential caused by the ions and molecules in the electrolyte. The electrode structure mimics that of a carbide-derived carbon (CDC) [14] , [15] and two different electrolytes were studied: the first consists of the pure ionic liquid 1-butyl-3-methylimidazolium (BMI + ) hexafluorophosphate ( ) at 400 K and the second of the same ionic species dissolved in acetonitrile (ACN), with a concentration of 1.5 M, at 298 K. As in our previous work, we use the coarse-grained models described in the Methods section for these liquids. These have been shown to reproduce their bulk and interfacial properties extremely well: in particular, we have shown that, when combined with the model porous carbons, this setup yields much higher capacitances than the ones obtained at planar electrodes [9] and in good agreement with experimental values. Although more accurate representation of the interactions could be used, at considerably enhanced computational cost, we note that the typical pore sizes of the carbon involved in the study are larger than the overall molecular sizes, so that a good representation of the interactions between the molecules and the pores should be achievable without capturing the full atomistic detail. Here the two systems exhibit integral capacitances of 87 F g −1 and 80 F g −1 , respectively, for an applied potential difference of 1 V between the two electrodes. Local structure characterization In order to characterize the local structure, we first use the simple concept of coordination number. As depicted in Fig. 1 , by defining a spherical cutoff distance R cut , it is possible to determine the number of a given molecular or atomic species coordinated to a central ion (note that R cut will be different from one pair to the other). Following the common practice, we defined R cut as the distance for which the corresponding radial distribution functions show a first minimum; the corresponding values are provided in Supplementary Table S1 . We further define a DoC for that ion as the percentage of the solid angle around the ion which is occupied by the carbon atoms [16] , normalized by the maximal value taken by this quantity (which would correspond to the hypothetical case of an ion encaged in a carbon sphere, see Supplementary Fig. S1 for more details). 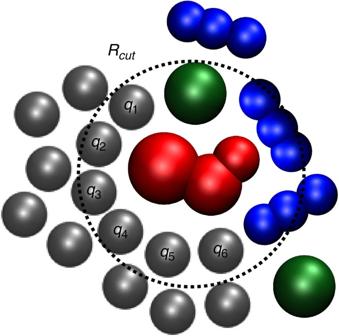Figure 1: Local structure characterization. Around each molecular ion, the number of neighbours of each species kind is determined using a spherical cutoff distanceRcut. In this example, the central cation (red spheres) is surrounded by one anion (green sphere) and two ACN (blue spheres) molecules. The local counter-charge on the electrode, which is the charge effectively stored, is simply determined by summing all the carbon atom (grey spheres) partial charges (in this example) and normalizing by the charge of one ion. The DoC is the percentage of the solid angle around the ion which is occupied by the carbon atoms, normalized by the maximal value taken by this quantity (seeSupplementary Fig. S1for details). Figure 1: Local structure characterization. Around each molecular ion, the number of neighbours of each species kind is determined using a spherical cutoff distance R cut . In this example, the central cation (red spheres) is surrounded by one anion (green sphere) and two ACN (blue spheres) molecules. The local counter-charge on the electrode, which is the charge effectively stored, is simply determined by summing all the carbon atom (grey spheres) partial charges ( in this example) and normalizing by the charge of one ion. The DoC is the percentage of the solid angle around the ion which is occupied by the carbon atoms, normalized by the maximal value taken by this quantity (see Supplementary Fig. S1 for details). Full size image The distributions of the DoC experienced by each ionic (BMI , ) or solvent (ACN) molecule adsorbed in nanoporous carbon electrodes held at null potential are shown in the upper panels of Fig. 2 . The values can differ markedly, ranging from 0% to 90%, and the occurrence of several broad peaks indicates that the molecules have some preferred DoC. By examining typical configurations, we have defined four different adsorption modes for the molecules: they can be lying close to (1) an edge site, that is, a carbon surface with a concave curvature, (2) a plane, which will have the local structure of a graphene sheet, (3) an hollow site, that is, a carbon surface with a convex curvature and (4) a pocket, when they are inside a subnanometre carbon pore with a cylinder-like shape (lower panel of Fig. 2 ). Of course, given the wide variety of atomic environments encountered in the CDCs, this limited classification necessarily simplifies the situation in the interest of assigning insight into the characteristic structures identified by the DoC measure. 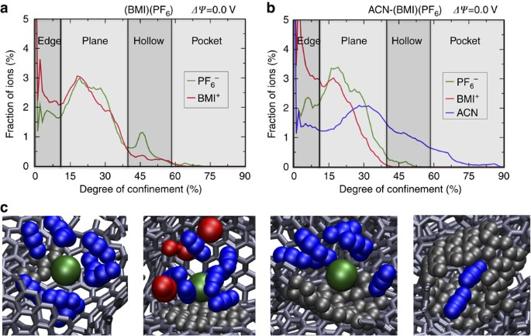Figure 2: Adsorption of the molecular species in a nanoporous carbon electrode at null potential. Upper panel: distribution of the DoC experienced by each ionic or solvent molecule in the pure ionic liquid (a) and in the ACN electrolyte (b). Four different adsorption modes are defined. Lower panel (c): representative configurations for each adsorption mode (grey rods, C–C bonds; red, BMI; green,; blue, ACN; grey spheres, C atoms which are in the coordination sphere of the central molecule). Figure 2: Adsorption of the molecular species in a nanoporous carbon electrode at null potential. Upper panel: distribution of the DoC experienced by each ionic or solvent molecule in the pure ionic liquid ( a ) and in the ACN electrolyte ( b ). Four different adsorption modes are defined. Lower panel ( c ): representative configurations for each adsorption mode (grey rods, C–C bonds; red, BMI ; green, ; blue, ACN; grey spheres, C atoms which are in the coordination sphere of the central molecule). Full size image For the pure ionic liquid, a majority of ions is located in edge and plane sites; a minority being adsorbed in hollow ones. The latter accept a larger number of anions than cations, which is consistent with their relative sizes. As for pocket sites, they are almost empty. On the other hand, for the ACN electrolyte, distinct behaviours are observed for the ionic species and the solvent molecules. Owing to their smaller size, the latter can easily be accommodated in small pores and a non-negligible number of ACN molecules are present in the pockets. Both BMI and ions in the ACN solution tend to lie on sites with lower DoC than in the pure ionic liquid. A few anions remain in hollow sites and the maximum of the distributions has moved to the edge site region for cations. This variation has two origins: First, the ions remain partly solvated in the ACN solution, which increases their effective size. Second, the filling of the smaller pores by the ACN molecules excludes them from these regions. Partial desolvation of the ions under confinement As expected from experimental studies [17] , [18] , the adsorption of ions in confined environments leads to their partial desolvation. This is clearly visible on the distributions of the ACN solvent molecule coordination number around each ion, as shown in Fig. 3 for (the data for the cations are provided in Supplementary Fig. S2 ). In the bulk electrolyte, this distribution is centred around 9, although occurrences of coordination numbers down to 4 and up to 14 are also observed. The more confined, the less solvated they become, with distributions centred around 8, 6–7 and 5–6 for edge, planar and hollow sites, respectively. In the case of pocket sites, it was not possible to extract such a distribution owing to the lack of statistics. Such a large desolvation effect has already been observed experimentally for aqueous solutions by Ohkubo et al . who have showed that Rb and Br hydration numbers decrease in slit-shape carbon nanospace by using extended X-ray absorption fine structure spectroscopy [19] . 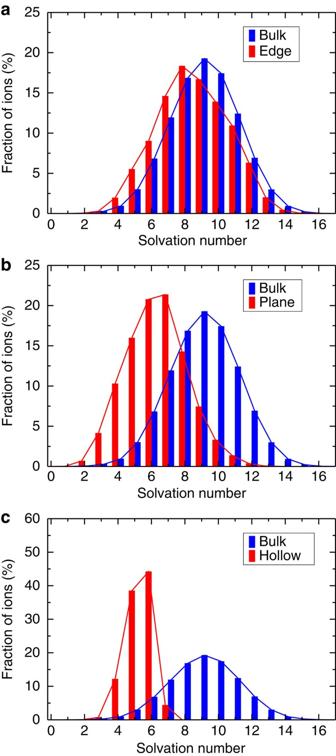Figure 3: Desolvation of anions in confined environment. Comparison of the ACN coordination number distributions around eachadsorbed on edge (a), planar (b) and hollow (c) sites (at null potential) and in the bulk electrolyte. Figure 3: Desolvation of anions in confined environment. Comparison of the ACN coordination number distributions around each adsorbed on edge ( a ), planar ( b ) and hollow ( c ) sites (at null potential) and in the bulk electrolyte. Full size image Effect of the electrode potential on the adsorption When a 1 V potential difference is applied between the electrodes, the number of ions in the electrodes and their DoC change drastically [9] . 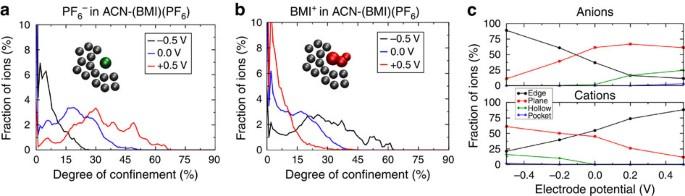Figure 4: Changes in the adsorption of the molecules with the electrode potential. Distribution of the DoC experienced by each(a) and BMI(b) for three different applied electrode potentials (−0.5, 0 and +0.5 V), in the case of the ACN-containing electrolyte. Variation of the fraction of ions adsorbed on edge, planar, hollow and pocket sites with the electrode potential (c). Figure 4 shows the variation of the DoC experienced by the ionic species (in the ACN electrolyte) inside electrodes at −0.5, 0 and +0.5 V, respectively. When passing from 0 to +0.5 V, anions are dragged towards the surface and they are less coordinated by cations and ACN. This permits them to enter into more confined pores, and ~30% of them are now adsorbed in the initially almost ions-free hollow and pocket sites. On the contrary, when the potential is decreased to −0.5 V, the few anions which remain inside the electrode occupy almost exclusively edge sites. A symmetrical behaviour is observed for the cations, as shown in Fig. 4 ; a striking point is that despite their relatively large size some of them are able to occupy pocket sites. This clearly shows that in addition to the already reported exchange of ions with the bulk [9] , the charging mechanism of supercapacitors involve drastic rearrangements in the distribution of ions inside the electrode, with a higher propensity for the ions charged oppositely to the electrode to adsorb in highly confined sites (note that similar patterns are observed for the pure ionic liquid, the corresponding plots are provided in Supplementary Fig. S3 ). In parallel, we also observe a further desolvation of the ions inside charged electrodes. In the case of hollow and pocket sites, some anions even become solvated by only a single ACN molecule (data provided in Supplementary Fig. S4 ), showing the strength of the interaction between the ions and the electrified carbon surface. Figure 4: Changes in the adsorption of the molecules with the electrode potential. Distribution of the DoC experienced by each ( a ) and BMI ( b ) for three different applied electrode potentials (−0.5, 0 and +0.5 V), in the case of the ACN-containing electrolyte. Variation of the fraction of ions adsorbed on edge, planar, hollow and pocket sites with the electrode potential ( c ). Full size image Our molecular dynamics simulations, performed using a realistic nanoporous carbon structure and allowing for the electrodes to be held at constant potential, provide a detailed picture of the local structure inside supercapacitors. At present, NMR seems to be the most promising experimental technique for probing the local structure inside supercapacitor electrodes. A system very similar to ours (that is, tetraethylammonium, TEA , and tetrafluoroborate, BF , ions dissolved in ACN and various CDC electrodes) was studied by probing the 11 B, 19 F and 1 H chemical shifts with increasing amounts of electrolyte [20] , [21] . In qualitative agreement with the present work, this study identified the presence of different environments for the confined BF ions, which could be assigned by increasing progressively the quantity of the electrolyte inside the CDC. For low loadings, only one peak is observed, which is thus assigned to ions which are adsorbed inside the nanopores. As the quantity of electrolyte increases, the intensity of this peak reaches a maximal value and a second peak is observed. The latter was assigned to anions which are in a confined liquid, that is, located in spaces between the primary particles of CDCs. Higher resolution may be possible in the future leading to specific sites being distinguished, which would allow a quantitative comparison with our simulations. Another recent NMR study focused on the same electrolyte ([TEA][BF 4 ] in ACN) [22] , but with activated carbon electrodes. Two adsorption modes were also observed; the authors attributed the first one to ions that sit between two graphene-like layers, whereas the attribution of the second one appeared more uncertain: the possibilities of adsorption on carbon rings made with five or seven carbons or on sites perpendicular to graphene planes were hypothesized by the authors. Although based on a different carbon microstructure, these results are also in qualitative accord with the picture proposed in Fig. 2 . Impact of the confinement on the local charge An advantage of our simulations is that they also provide us with the instantaneous charge carried by each carbon atom. It is therefore tempting to see how the local surface charge depends on the adsorption mode. We have performed such an analysis by calculating the counter-charge on the electrode per adsorbed ion as schematized in Fig. 1 : we calculate the sum of the charges of the carbon atoms located at distances smaller than R cut around a given ion and normalize this quantity by the charge of the ion. It is plotted with respect to the DoC in Fig. 5 for two applied potentials (0 V and 1 V) in the case of the ACN-based electrolyte (similar trends are obtained for the pure ionic liquid, the corresponding data are provided in Supplementary Fig. S5 ). At null applied potential, the total charge on the electrode oscillates around zero, but locally the carbon atoms can carry a charge: the resulting local charge appears to be completely correlated to the nature of the nearby adsorbed ions, which determine its sign, and to the DoC of the latter. The net counter-charge near ions in edge sites is close to 0 e, whereas higher values (up to 30% of the ionic charge) are obtained in plane and hollow sites. In these cases, the largest charge on an individual carbon atom was 0.03 e. For an applied potential of 1 V, a similar trend is obtained but, owing to the higher occupation of hollow and pocket sizes, much larger local charges are observed. We note again a qualitative agreement with the experimental results of Vix-Guterl et al . [23] , who have observed a linear dependence between the capacitance and the ultramicropores volume (but for different porous carbon/electrolyte combinations). It is worth noting that in the positive (negative) electrode, the local counter-charge close to cations (anions) is positive (negative). It is important to bear in mind that even if the analysis performed here is based on the characterization of the local surface close to a given ion, on the liquid side of the interface other counterions, co-ions (in smaller quantity [9] ) and solvent molecules are also present and influence the local counter-charge on the electrode. 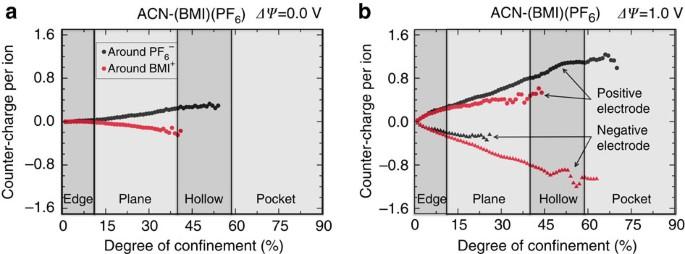Figure 5: Effect of confinement on the efficiency of charge storage. The counter-charge on the electrode per adsorbed ion, calculated as schematized inFig. 1is plotted versus the DoC of the ion, for applied potentials of 0 V (a) and 1 V (b) in the case of the ACN-based electrolyte. Figure 5: Effect of confinement on the efficiency of charge storage. The counter-charge on the electrode per adsorbed ion, calculated as schematized in Fig. 1 is plotted versus the DoC of the ion, for applied potentials of 0 V ( a ) and 1 V ( b ) in the case of the ACN-based electrolyte. Full size image The DoC (or conversely the extent of decoordination/desolvation of the ion) has a substantial impact upon the local charge stored on the electrode surface and indicates some key directions for the optimization of materials for supercapacitors. This result confirms the numerous recent electrochemical studies in which an increase of the performance was observed in such materials [5] , [6] , [23] , [24] . From the theoretical point of view, the main effects responsible for the origin of the enhancement of the capacitance with porous electrodes were already established, that is, the electronic screening by the pore walls of the repulsive Coulombic interactions between ions of the same charge and the absence of overscreening effects in the electrolyte [9] , [10] , [11] . This work now goes further by demonstrating unambiguously the key role of the local structure and by revealing the role of coordination and solvation. In qualitative agreement with recent NMR studies, we have shown that the absorbed ions can partition themselves among different adsorption sites in a way which depends on the applied potential [20] , [21] , [22] and we have detected four different sites in the case of a given CDC. Depending on the number of carbon atoms which lie in their vicinity, we distinguish edge sites (concave curvature), plane sites (graphene sheet-like structure), hollow sites (convex curvature) and pocket sites (inside a subnanometre carbon pore). In parallel, the local charge stored at the surface of the electrode increases as the DoC of the adsorbed ions increases. Although it was observed from experiments and some simulations that the best performances were obtained for CDCs with an average pore size matching the size of the ions [24] , [25] , [26] , [27] , [28] , in a recent theoretical study, Kondrat et al . [29] have shown that the best average pore size depends on the operating voltage. Nevertheless their model was based on a description of the porous carbon based on a distribution of slit-like pores; the present results show that it would be necessary to inject a more detailed adsorption model to fully address this point. It is also probable that the different adsorption sites will have different behaviour from the dynamic point of view, which may impact the power performances of the device [30] . These results are not only important from the fundamental but also from the practical point of view. Nanoporous carbons may be synthesized by numerous routes, resulting in a huge variety of local structures which differ by their pore size distribution, the presence of defects and so on. The development of spectroscopic techniques may open the possibility for characterizing further the structures on the local scale, and the combination of such data with our simulation results would then allow for the controlled optimization of electrode/electrolyte couples, for example, by choosing directly the best-adapted electrolyte for a given carbon structure. Molecular dynamics simulations The simulation cells consist of an electrolyte surrounded by two porous carbon electrode ( Supplementary Fig. S6 ). The ions and molecules of the two electrolytes considered are represented by a coarse-grained model in which the cations and ACN molecules are made of three interaction sites and anions are rendered by a single interaction site [31] , [32] . All the force field parameters, including the interactions between electrolyte species and carbon atoms can be found in our previous work [33] . The coarse-grained model was developed in order to yield the correct thermodynamic and transport properties of the bulk liquids [31] , [32] . Note that for the ions, we use the revised version of the force field by Roy and Maroncelli, for which the calculated diffusion coefficients match very well the experimental ones on a wide range of temperatures. This model has also been tested in previous simulations involving interfaces with carbon electrodes both for the pure ionic liquid [34] and for solutions in ACN [33] . The results show that the structure of the liquid at the interface and the capacitive properties of the system are in very good agreement with other simulations conducted with all-atom models. The details of the simulation cells are provided in Supplementary Table S2 . The carbon structure for the porous electrodes was obtained through quenched molecular dynamics [15] and corresponds to the experimental structure of a CDC synthesized at 1,200 °C, with an average pore size of 0.9 nm. As in our previous works [9] , [13] , where we showed that it is essential to include electrode polarizability, we model the carbon electrode as a perfect conductor. A fixed potential difference is imposed between the positive and negative electrodes. The charges are determined at each time step so as to enforce the constant potential condition. Although this methodology is the state of the art in current simulations of supercapacitors [33] , we note recent works in which it was shown that the perfect conductor character could be affected by the effects of field penetration [35] . Further simulation work involving more complex models for the electrodes will therefore be tested in the future [36] , although this is probably not feasible for the moment owing to the high computational cost involved for the large porous electrodes. The simulations are conducted in the NVT ensemble with a timestep of 2 fs which is consistent with the coarse-grained model used. The temperature is maintained at 400 K for the pure ionic liquid and 298 K for the ACN electrolyte by applying a Nosé–Hoover thermostat with a time constant of 10 ps. Two-dimensional periodic boundary conditions are used, that is, there is no periodicity in the direction perpendicular to the electrodes, and the Ewald summation is adapted to this set-up [37] , [38] . A special procedure is used to acquire initial configurations for the production runs. The simulations cells are ‘charged’ and ‘discharged’ a first time before starting equilibration runs. This is done by setting the charges of each carbon atom of the carbon electrodes equal to 0.002 e for 100 ps and then changing their values back to 0 e. This results in a better filling of the porous electrodes compared with neutral conditions only. The system is then further equilibrated during 1.3 ns with a constant charge of 0 e on the carbon atoms. During the last nanosecond of this equilibration run, configurations are extracted every 100 ps and used as starting points for the production runs at 0.0 V. Following the same procedure, the system is equilibrated during 1.3 ns with constant charges equal to −0.01 e and +0.01 e on the carbon atoms and configurations are extracted during the last nanosecond to acquire starting configurations for the production runs at 1.0 V. For each potential difference, 10 production runs of 20 ps each are conducted leading to a total of 200 ps of constant potential simulations. Definition of the DoC We define the DoC as the percentage of the solid angle around ions which is occupied by carbon atoms, normalized by the maximal value taken by this quantity. For a given ion i , the solid angle associated with a carbon atom j , located at a distance from this ion, is given by [16] : where is the radii of the region occupied by . In the porous electrodes modelled in this work, most of the carbon atoms are part of cycles comprising six carbon atoms. As a consequence, the carbon–carbon distance is nearly constant and equal to 1.43 Å. Thus, it seems adapted to choose equal to half of this carbon–carbon distance. For a perfectly dense system, the total solid angle around a given ion can reach the maximal value of 4 . But, as depicted in Supplementary Fig. S1 , for graphitic structures, the cycle surface is not completely covered by the carbon atoms. A quick geometrical examination shows that only 60.46% of the surface is effectively covered. With these considerations, we now write the DoC for a given ion as follows: where CN is the carbon coordination number around ion . How to cite this article: Merlet, C. et al . Highly confined ions store charge more efficiently in supercapacitors. Nat. Commun. 4:2701 doi: 10.1038/ncomms3701 (2013).